A new regime for mechanical annealing and strong sample-size strengthening in body centred cubic molybdenum Because of crystal symmetry, body centred cubic (BCC) metals have large differences in lattice friction between screw and edge dislocations, and manifest generally different mechanical behaviours from face centred cubic (FCC) metals. Although mechanical annealing (significant drop in stored dislocation density in response to applied stress) has been observed in FCC metals, it has not been observed in BCC metals so far. Here we show that significant mechanical annealing does occur in BCC Mo pillars, when their diameters decrease to hundreds of nanometers. In addition, there exists a critical diameter for focused ion beam milled pillars, below which the strengthening exponent increases dramatically, from ~0.3 to ~1. Thus, a new regime of size effects in BCC metals is discovered that converges to that of FCC metals, revealing deep connection in the dislocation dynamics of the two systems. The deformation behaviour of small-volume metals, in particular the effects of sample size (that is, the diameter D of micro- and nano-pillars) on the apparent strength σ , has been attracting considerable attention recently [1] , [2] , [3] , [4] , [5] , [6] , [7] . A number of studies of single-crystal micro- and nano-pillars have demonstrated the 'smaller is stronger' trend, with the flow stress increasing markedly with decreasing sample size. The strength appears to follow an empirical power law [8] , scaling with D as D − α . Although it is generally believed that dislocation source limitation is responsible for the D dependence [7] , [9] , [10] , [11] , the exact origin of the size effect remains a subject of intense debate [8] . Particularly interesting are the behaviours of BCC metals, which in bulk form tend to exhibit significant deviations from FCC metals. Molybdenum (Mo) is a representative and widely studied example [3] , [4] , [5] , [6] , [12] , [13] , [14] of such BCC metals. The behaviour of Mo pillars is intriguing in two aspects. First, investigations so far indicate BCC Mo pillars exhibit a relatively weak sample-size dependence at room temperature [3] , [15] , [16] . In an extreme case of Mo-alloy pillars produced by high-temperature eutectic solidification followed by chemical etching, the samples were believed to be initially dislocation free, and the flow stress was reported to be independent of the pillar size [4] , [17] . In focused ion beam (FIB) micro-machined pillars, α was found to be <~0.45 for Mo by several groups [3] , [15] , [16] , considerably lower than those for FIBed FCC metallic pillars. This major difference has been postulated to be related to the known difference in the mobility of screw dislocations. The Peierls barrier of screw dislocation is much higher than those of non-screw dislocations in BCC metals, so the mobility of screw dislocation is exceptionally low and strain rate-controlling in conventional plasticity of BCC metals [18] , whereas, in FCC metals, the Peierls barrier is low as well as similar for screw and non-screw dislocations [19] , [20] , [21] . It is known that the athermal shear stress for screw dislocation motion in Mo is 750 MPa (the corresponding uniaxial stress would be of the order of 1.5 GPa) near 0 K (ref. 22 ). At stresses far above this level, such that the free-flight dislocation velocity is exceedingly high, for example, approaching the speed of transverse acoustic wave, the mobility difference between edge and screw dislocations is expected to diminish. This trend was confirmed by our molecular dynamics (MD) simulation. 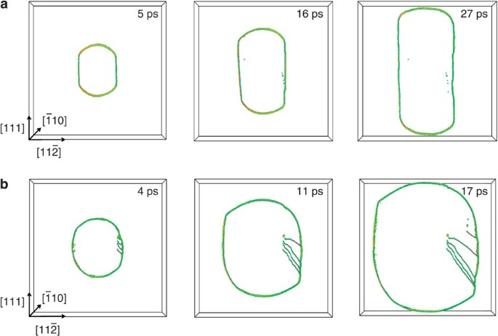Figure 1: Effect of stress level on dislocation loop expansion at 20 K from MD simulations. (a) The loop developed into a track-field-like geometry when the external applied shear stress was fixed at 1.5 GPa, consistent with the traditional understanding that screw dislocations move much slower than edge dislocations. (b) When the externally applied shear stress was increased to 4 GPa, the dislocation loop kept a roughly round shape during its expanding process. This means that the mobility of the screw and edge segments now becomes similar under such high stresses. As shown in Figure 1 , a dislocation loop developed into a track-field-like geometry, when the external applied shear stress was fixed at 1.5 GPa. However, when the externally applied shear stress was increased to 4 GPa, the dislocation loop kept a roughly round shape instead during its expansion. According to the tenet of 'smaller is stronger', for sufficiently small pillar size and, therefore, high enough prevailing stress, the dislocation dynamics and, hence, the size dependence in BCC metals could become more similar to that in FCC pillars. Figure 1: Effect of stress level on dislocation loop expansion at 20 K from MD simulations. ( a ) The loop developed into a track-field-like geometry when the external applied shear stress was fixed at 1.5 GPa, consistent with the traditional understanding that screw dislocations move much slower than edge dislocations. ( b ) When the externally applied shear stress was increased to 4 GPa, the dislocation loop kept a roughly round shape during its expanding process. This means that the mobility of the screw and edge segments now becomes similar under such high stresses. Full size image Second, mechanical annealing has not been experimentally observed in Mo pillars [23] , even though the concept of mechanical annealing does not contradict Weinberger and Cai's simulation in which a single screw dislocation can be pushed out of the pillar without self-breeding at lower stresses (<5.5 GPa in D =36 nm pillar) [5] . Mechanical annealing [24] refers to the reduction of dislocation density in the deforming volume, when dislocation generation and accumulation is outweighed by dislocation annihilation and escape from the surfaces. For FCC pillars below a certain D C , mechanical annealing renders the pillar almost dislocation free [24] . In contrast, in Mo pillars, it has been shown that dislocation tangles are retained even after extensive plastic deformation [23] . This has been rationalized by MD simulations of Mo pillars as due to dislocation self-multiplication at higher stresses (>5.5 GPa in D =36 nm pillar), arising from the cross-kinks generated along the screw dislocations that have non-coplanar core structure [5] , [14] . Many in the community believe that mechanical annealing is not possible for BCC metals regardless of sample size. In this work, we investigate these two issues by in situ transmission electron microscope (TEM) compression of FIBed Mo pillars over a wide D range that includes smaller sizes than those accessed before. We uncovered three different stress regimes, in which explosive dislocation nucleation through dislocation self-multiplication (high-stress regime, HSR), mechanical annealing (medium-stress regime, MSR) or bulk-like plasticity (low-stress regime, LSR) dominates, respectively. We also demonstrate and explain that there is a marked change in α not only for BCC versus FCC pillars, but also for BCC pillars in different D regimes. 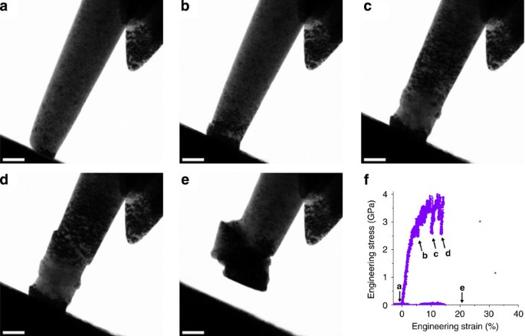Figure 2: Mechanical annealing during thein situnanocompression test of a typical Mo nanopillar. Bright-field TEM images of the diameterD=142 nm pillar before (a) and after (e) thein situcompression test. (b), (c), (d) and (e) correspond to the marked points in the engineering stress versus strain curve in (f). The scale bar in each figure represents 100 nm. See also the recorded video inSupplementary Movie 1. Mechanical annealing in Mo Figure 2 shows one typical example of the <111> oriented pillars. In this case, the starting pillar had D ~142 nm at the free end, 660 nm in height and a sidewall taper angle of about 4° with a high density of FIB-induced surface defects ( Fig. 2a ). The TEM bright-field images here, Figure 2a through Figure 2e , are still frames extracted from the movie recorded during the nanocompression test, in one-to-one correspondence with the five points (a through e) marked in its engineering stress versus strain curve displayed in Figure 2f . In this work, the engineering stress was defined as the instantaneous force divided by the smallest cross-sectional area just before the structural collapse. Admittedly, this will underestimate the stress before the collapse point. For example, if we plot the instantaneous contact stress versus strain, there will be no more 'strain hardening' ( Supplementary Fig. S1 ). However, this convention will make sure the collapse stress is always the true stress, which is the main focus of this work. Figure 2: Mechanical annealing during the in situ nanocompression test of a typical Mo nanopillar. Bright-field TEM images of the diameter D= 142 nm pillar before ( a ) and after ( e ) the in situ compression test. ( b ), ( c ), ( d ) and ( e ) correspond to the marked points in the engineering stress versus strain curve in ( f ). The scale bar in each figure represents 100 nm. See also the recorded video in Supplementary Movie 1 . Full size image Dislocations were found to emerge from the contact interface (heterogeneous dislocations sources) between the pillar and the punch, and accumulate near the free end even before the apparent 'yield' point b in Figure 2f , in LSR. Beyond this point (that is, getting into MSR), the ensuing plastic deformation cleans up the dislocations in the regions near the free end, except at the location in immediate contact with the interface. Presumably, this is due to the friction confinement between the diamond tip and the pillar. Apparently, mechanical annealing did occur and continued through stages c and d. Serrations are obvious in the curve (for example, at points c and d in Fig. 2f ). They are due to intermittent shear along certain slip planes in the 'cleaned up' region, a phenomenon often seen during the plastic flow in small pillars. The stress is observed to reach a value near 4 GPa (HSR) before the structural collapse at point d. The evolution of the pillar together with the responsible dislocation activities can be better visualized in Supplementary Movie 1 . The cleaned region ( Fig. 2d ) after mechanical annealing looks rather like the pristine Mo achieved by high-temperature formation or annealing [4] , [12] , in the sense of lacking 'obvious' dislocation lines ('obvious' defined here by the contour length of a dislocation being a significant fraction of D ) or dislocation forest inside. But one cannot tell whether some point defects or tiny point-defect clusters still remain in the cleaned region, as they are beyond the resolution of conventional TEM. It is quite likely that mechanical annealing can only achieve partial cleaning-up compared with bona fide high-temperature thermal annealing. Certainly, Ga solutes may escape as gas during high-temperature thermal annealing, but unlikely to do so during mechanical annealing, so the chemical implantation induced by FIB is unlikely to be cleaned away by mechanical annealing. Consequently, our mechanically annealed region is still not as structurally perfect as the high-temperature processed pillars near the melting point [4] , [17] , and the strong size dependence of the collapse strength is consistent with that. The subsequent collapse of mechanically annealed region ( Fig. 2d,e ) and those in previous works [4] , [12] may result from the onset of the dislocation self-multiplication as described in ref 5 . However, it is worth noting that the predicted critical stress in ref 5 . for smaller pillars (with obvious mechanical annealing observed experimentally) marks the upper bound instead of lower bound of the measured strength. This is because the dislocation density (after mechanical annealing) falls on the left side of the saddle point in the stress versus dislocation density curve [25] . In short, the starting material (FIBed pillar) contained high density of defects and the stress was ramped up gradually. The time sequence was LSR → some dislocation breeding by surface emission and Frank-Read mechanism ( Fig. 2b ) → MSR → mechanical annealing ( Fig. 2c,d ) → dislocation-free region created in Figure 2d (no 'obvious' dislocations in the region) → HSR → the dislocation-free region collapsed by explosive dislocation self-multiplication → the system unloaded and passed through MSR to LSR. However, the system unloaded very quickly and spent very little time in MSR. In thermal annealing, the annealing time (typically minutes to hours) is as important as the annealing temperature. If the time-at-temperature is very short, it is quenching instead of annealing, and quenching preserves defects. The same is true for mechanical annealing: because of the high stress-quench rate, there is insignificant mechanical annealing, so the system unloaded to zero stress ( Fig. 2e ) with a lot of quenched-in dislocations as 'fossil record' of the HSR explosive dislocation self-multiplications. Strong sample-size strengthening Similar behaviour of mechanical annealing and eventual structural collapse was repeatedly observed in other Mo pillars with D <200 nm. Another example is the D =80 nm pillar shown in Supplementary Figure S2 (see also Supplementary Movie 2 ). 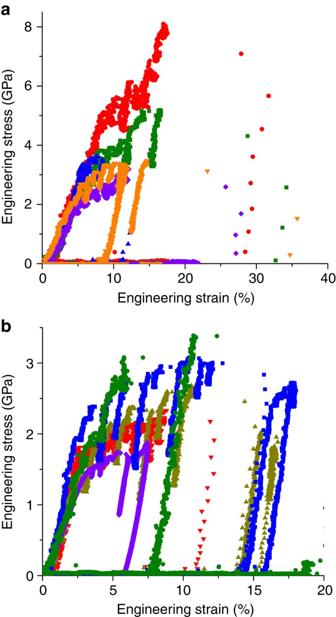Figure 3: Representative engineering stress–strain curves of Mo nanopillars. (a) DiameterD<200 nm, including 80 nm (red), 120 nm (green), 165 nm (blue), 172 nm (orange) and 185 nm (purple). (b) DiameterD>200 nm, including 268 nm (green), 369 nm (blue), 463 nm (yellow), 607 nm (red), and 1,200 nm (purple). For this group of pillars, their representative engineering stress-strain curves are displayed in Figure 3a . For comparison, the curves for D >200 nm pillars are displayed in Figure 3b where discrete strain bursts are also noticeable, consistent with previous reports on similar-sized Mo pillars by Greer et al . [3] , [13] , [14] and Arzt et al . [6] , [16] But due to their larger sizes, mechanical annealing should be less obvious; or rather, the effect of mechanical annealing is counterbalanced by dislocation creation inside by more traditional means (for example, Frank-Read sources). Figure 3: Representative engineering stress–strain curves of Mo nanopillars. ( a ) Diameter D <200 nm, including 80 nm (red), 120 nm (green), 165 nm (blue), 172 nm (orange) and 185 nm (purple). ( b ) Diameter D >200 nm, including 268 nm (green), 369 nm (blue), 463 nm (yellow), 607 nm (red), and 1,200 nm (purple). 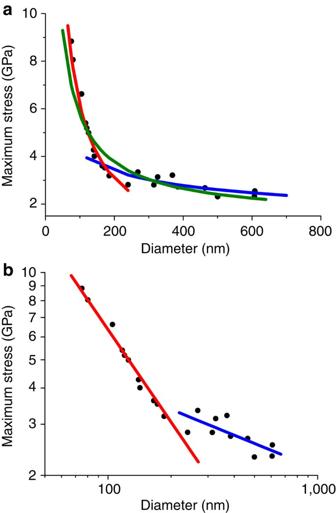Figure 4: Sample-size strengthening of Mo nanopillars. (a) Maximum flow stress before collapse plotted as a function of pillar diameterD(black dots), showing two regimes with apparently differentDdependences (power law fits without consideringσ0; see blue and red lines for larger and smaller diameter regimes, respectively). Green line is the fit of experimental data using equation (1). (b) Double-log plot showing two differentαvalues, 1.0 and 0.29 for red and blue lines, respectively. Full size image The maximum flow stress sustainable in each pillar before the final collapse, σ f , is plotted in Figure 4a as a function of D . An obvious sample-size effect is observed, with σ f clearly increasing with decreasing D . There appears to be two size regimes, corresponding to the two groups of pillars in Figure 3a,b . For the group with D >~200 nm, the D dependence of σ f is relatively weak. Plotting log σ f versus log D , we obtain the slope α ~0.3, as shown in Figure 4b . This α is consistent with that found in previous reports ( α =0.22 to 0.45, for a similar D -range [3] , [15] , [16] ). In contrast, a dramatically different slope (about 3 times larger) is observed when the pillar sizes were reduced to below D C =200 nm. Similar trend was obtained, if the flow stress values were taken at a fixed strain (for example, at 5% strain, as done by some groups for other metal pillars [15] ). The relatively low data scatter of the σ f of our smaller pillars (<~200 nm), where mechanical annealing reduced dislocation density down to ~0, seems to be consistent with the previous observation that dislocation-free crystals tend to show smaller data scatter [17] , [26] , [27] . Figure 4: Sample-size strengthening of Mo nanopillars. ( a ) Maximum flow stress before collapse plotted as a function of pillar diameter D (black dots), showing two regimes with apparently different D dependences (power law fits without considering σ 0 ; see blue and red lines for larger and smaller diameter regimes, respectively). Green line is the fit of experimental data using equation (1). ( b ) Double-log plot showing two different α values, 1.0 and 0.29 for red and blue lines, respectively. Full size image The dramatic rise in α indicates that the size-strengthening of FIBed Mo pillars is much more pronounced below a transition size ( D C ~200 nm) than that reported for larger pillars [3] , and that the size-dependence itself also has a strong size effect; in other words, the degree of size-strengthening can be very different in distinctly separable D regimes. It appears that for sufficiently small BCC Mo pillars, the size-strengthening becomes FCC-like, just as the FCC-like mechanical annealing discussed earlier. In the following, we present a simple analysis to rationalize the two seemingly different regimes, and explain the previously noted difference between BCC and FCC metals [15] . For the different α , previous arguments invoked the difference in screw dislocation mobility through the lattice as the possible cause [15] . However, they do not explain exactly how this would result in a α much smaller for BCC metals than for FCC metals. Also, as noted earlier, for very small Mo pillars, the prevailing stresses are far above the athermal threshold stress for single screw motion; this would partly diminish the difference in the mobility of screw and edge dislocations as discussed in Figure 1 . In general, the observed strength is not simply controlled by lattice friction to dislocation motion. Instead, to match the imposed strain rate, the dislocations need to multiply, similar to the dislocation source limited deformation in small-volume FCC pillars. As shown by Weinberger and Cai [5] for BCC Mo, at sufficiently high stresses above a critical stress, σ c , the cross-kink debris (loops) left behind the moving screw dislocations can open up, becoming sources of dislocations themselves. This self-multiplication overwhelms the annihilation (mechanical annealing), resulting in an outburst of dislocations to mediate the dramatic shape change ( Fig. 2e ), that is, the collapse. The HSR–MSR boundary σ c is therefore the σ f plotted in Figure 4 . σ f can be modelled by modifying the σ c expression of Weinberger et al . [5] into Here σ 0 is the lattice friction contribution to flow stress from screw dislocation's high-speed motion through the lattice accompanying the sample collapse. σ 0 is taken to be 1.3 GPa, which is almost the same as the average yield stress for 4% pre-strained Mo pillars with size of ~1,200 nm and the flow stress for 11% pre-strained Mo pillars regardless of pillar diameter [17] . The second term, which brings in the D dependence, is the stress needed for the dislocation to execute self-multiplication by bow-out [5] , which becomes operative at HSR in lieu of the double-kinks mechanism. Here G is the shear modulus; b is the Burgers vector. The source size is assumed to scale with D , and the scaling factor is accounted for by the fitting parameters, β and B . The fit using equation (1), as shown by the green line in Figure 4a , represents the experimental data fairly well, and gives β =1.83 and B= 0.109 nm. At very small D , the second term in the bracket in equation (1) is much larger than unity, such that the former can be dropped. In this case, in a log σ f –log D plot, the D dependence is governed by the 1/ D term, giving α ~1. In other words, σ 0 is only a small part of the very high σ f for these small pillars such that the effective D -sensitivity is large. In contrast, when D is relatively large, σ 0 becomes a significant part of the σ f so that the effective D -sensitivity gets weaker. If one then continues to assume a D − α power law (in lieu of equation (1)), the slope in a log σ f −log D plot would give an effective α significantly lower than 1 ( α ~0.3 in Fig. 4b ). Therefore, the general size dependence, equation (1), can be approximated by two size regimes represented by two different simple power-law dependences on D , as shown in Figure 4b . The two corresponding power-law fits to the σ f − D data are drawn in Figure 4a , exhibiting the different D sensitivities as expected. The magnitude of σ 0 does make a difference in controlling the apparent α , even when the observed strength is actually mostly dislocation-source-controlled. The large magnitude of σ 0 for BCC Mo renders the second size regime (weaker D dependence) obvious, once the D surpasses a couple of hundred nanometers. In comparison, for FCC metals σ 0 is known to be much smaller [18] . As a result, the D dependence remains stronger for a large D range. The same is also true for some BCC metals such as Nb, for which room temperature is already close to the critical temperature [28] at which thermal fluctuation energy can overwhelm the Peierls barrier to produce a relatively small σ 0 . Figure 1 shows that simply reaching the athermal threshold or even σ 0 is not enough to eliminate the mobility difference between the screw and edge dislocations. This is because the latter is fully accomplished only in the limit that the dislocations possess velocities approaching the transverse acoustic wave velocity, thus requiring extraordinarily high stresses near the ideal strength; at lower velocities and stresses, the screw dislocations always possess mobility advantage owing to their non-planar cores. Therefore, the transition to become FCC-like requires a very small size (for example, D< ~200 nm), when the stress eventually reaches sufficiently high levels. Sample preparation The starting material we used was a directionally solidified bulk Mo single crystal. The as-received crystal was ~10 mm in diameter and 3 mm in height, with the axis along <111> direction. Several pieces of samples with their dimension of 0.5 mm×2 mm×2.5 mm were cut by electric-discharge machining with the edge of the length direction oriented along <111> direction. The samples were then mechanically thinned to 0.05 mm in thickness and subsequently electro-polished at the middle part of a selected edge (2.5 mm) using a solution of 60% Methanol, 35% 1-Butanol and 5% HClO 4 . One selected sample was then mounted carefully onto a copper substrate used for in situ TEM nanocompression test. The edges (2 mm) of the sample was aligned carefully so that the axis of those later fabricated pillars will be the <111> crystal orientation. More details about the sample preparation method are described in the work by Shan et al . [24] The FIB cutting in this work was performed through three steps, from rough machining to fine milling and eventually to final superfine polishing, as illustrated in Supplementary Figure S3a–c . The beam current was reduced to 1.5 pA at the last milling step to minimize FIB damage. Pillars with diameters from 75 to 1,200 nm were obtained with their taper angles ranging from 2 to 4.5° The systematic variation of pillar diameter allows the determination of the sample-size dependence of strength in the nanoscale regime not accessed in previous studies. The final diameters and heights of the pillars were measured using s.e.m. Experimental methods In situ compression tests were performed in a JEOL JEM-2100F TEM using the Hysitron PI95 PicoIndenter with a flat diamond punch (tip diameter ~1 μm). The compression tests were conducted at a constant displacement rate in the range of 2 to 5 nm s −1 . The engineering stress σ was calculated as σ =4 F / πd 2 , where F is the measured force and d is the contact diameter before collapse. The engineering strain ɛ was calculated as ɛ =Δ L / L 0 , where Δ L is the compression displacement and L 0 is the initial pillar height. MD simulation methods Large scale parallel molecular dynamics program LAMMPS [29] and visualization program AtomEye [30] were employed to perform the simulations and visualization. Finis–Sinclair potential [31] was used to describe the atomic interaction of molybdenum atoms. The computational supercell had the dimensions , , z =180×[111] with periodic boundary condition in x and z directions and free surface in y direction. Dislocation loop with Burgers vector b =1/2[111] was introduced by shifting the upper slab with respect to the lower slab by a Burgers vector along z direction and was relaxed by conjugate gradient relaxation method. All simulations were carried out under the NPT (constant atom number, external pressure and temperature) ensembles with temperature T =20 K, P xx =0.0 GPa and P zz =0.0 GPa. Shear stress τ yz was realized through adding a constant force to each atom in the several atomic layers of upper and lower free surface. A time step of 1 fs was used during the integrating of Newton's equation of motion. How to cite this article: Huang, L. et al . A new regime for mechanical annealing and strong sample-size strengthening in body centred cubic molybdenum. Nat. Commun. 2:547 doi: 10.1038/ncomms1557 (2011).